Flutter-driven triboelectrification for harvesting wind energy Technologies to harvest electrical energy from wind have vast potentials because wind is one of the cleanest and most sustainable energy sources that nature provides. Here we propose a flutter-driven triboelectric generator that uses contact electrification caused by the self-sustained oscillation of flags. We study the coupled interaction between a fluttering flexible flag and a rigid plate. In doing so, we find three distinct contact modes: single, double and chaotic. The flutter-driven triboelectric generator having small dimensions of 7.5 × 5 cm at wind speed of 15 ms −1 exhibits high-electrical performances: an instantaneous output voltage of 200 V and a current of 60 μA with a high frequency of 158 Hz, giving an average power density of approximately 0.86 mW. The flutter-driven triboelectric generation is a promising technology to drive electric devices in the outdoor environments in a sustainable manner. As the needs for the portable and wireless electronics have been growing rapidly, the energy-harvesting technology has been highlighted as a promising solution to supply the electrical power without wiring to external sources. So far, diverse environmental energy sources have been exploited for the energy harvesting, such as mechanical vibration, light, heat and electromagnetic radiation. Among possible environmental energy sources, wind energy can be an ideal source for energy-harvesting system due to its absolute abundance [1] , [2] , [3] and has long been actively developed since the invention of the windmill. Recently, flow-induced vibration of flexible structures has been suggested as an alternative to overcome the drawbacks of wind-turbine-based wind energy generator including structural complexity, the large volume and weight, high cost of manufacturing and installation, low efficiency and noise. Most research in this area is focused on piezoelectric materials [4] , [5] , [6] , [7] such as lead zirconium titanate and polyvinylidene fluoride, where a deformation of piezoelectric material gives rise to electrical energy. The recently invented triboelectric generator harvests mechanical energy through a periodic contact motion based on the coupling of the triboelectric and electrostatic effects, and many approaches have been carried out to improve the electrical output performance of the triboelectric generator [8] , [9] , [10] , [11] , [12] , [13] , [14] , [15] , [16] . A triboelectric generator is one of the most promising energy conversion systems due to its low cost, simple fabrication routes and the possibility of high-power density [17] , [18] . Meanwhile, there has been considerable research on the basic dynamics of flexible structures like flags, which can be bent, folded, twisted or waved in the air [19] , [20] , [21] , [22] , [23] , [24] , [25] , [26] . The first experimental study on fluttering behaviour was performed by Taneda [27] with a flag made of various fabrics and shapes, to find a variety of flapping modes (for example, nodeless, one-node, imperfect-node and two-node flutters). In addition, using one-dimensional filaments, the distinct dynamic states (for example, a stretched-straight state and a flapping state) and the coupled interaction between the states were observed through a flowing soap film experiment [28] . On the other hand, the interaction of the flag and a counter rigid plate hitherto has received scant attention, although their coupled dynamics can be a very powerful vibration source for triboelectric generator due to its self-sustained nature. In the present work, we first investigate the interaction dynamics of a flexible flag textile and a solid plate to obtain the stability boundaries of fluttering. We show that the dynamic behaviours can be classified into three distinct regimes of single contact, double contact and chaotic contact. We then develop a flutter-driven triboelectric generator (FTEG), consisting of a flag and a counter plate arranged in parallel with respect to the air stream, based on the knowledge of the interaction dynamics of the flag and plate. As a result, the instantaneous output voltage, current and power of 7.5 × 5-cm size FTEG reaches 250 V, 70 μA and 17.5 mW, respectively, at the incoming flow velocity of 22 ms −1 . In addition, the frequency of the electrical signal is extremely high (about 115 Hz) compared with the previously suggested energy-harvesting devices [15] , which ensures the overwhelming electrical performance of the current FTEG. The 7.5 × 5-cm size FTEG with a dual-plate configuration at the incoming air velocity of 15 ms −1 can fully charge a 100-μF capacitor within 4 min. In ambient open environment, we demonstrate that the FTEG can be easily developed for the large-scale energy-harvesting system as well, with an extremely simple fabrication process, very low cost and weight. Flutter-driven triboelectric generator set-up For the construction of the simplest wind-driven energy-harvesting system using fluttering behaviour, a flexible flag and a rigid plate were arranged in face to face as shown in Fig. 1a so that the interaction between them can lead to a rapid periodic contact and separation. The flexible flag with a metal coated on the surface acts as the fluttering body as well as an electrode. Polytetrafluoroethylene (PTFE), a triboelectric material of high electron affinity, was attached to the surface of the rigid plate to achieve contact electrification between conductor and dielectric. The two structures become oppositely charged whenever they are in contact. The subsequent separation of the two charged structures induces an electronic potential difference that can induce the flow of free electrons to an external circuit. This simple mechanism can be successfully employed for converting the kinetic energy of the wind to electrical energy. 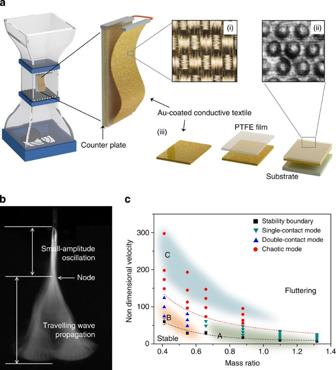Figure 1: Experimental set-up and characterization of fluttering behaviour. (a) Schematic diagrams of a wind tunnel and the structural design of a flutter-driven triboelectric generator including surface characteristics of (i) a highly flexible flag and (ii) a counter plate and (iii) the fabrication of the counter plate. (b) Fluttering images of a stand-alone configuration of dimensions 7.5 × 5 cm as captured with a high-speed camera. (c) The regime map of the dynamic interaction between a flag and a plate. Figure 1: Experimental set-up and characterization of fluttering behaviour. ( a ) Schematic diagrams of a wind tunnel and the structural design of a flutter-driven triboelectric generator including surface characteristics of (i) a highly flexible flag and (ii) a counter plate and (iii) the fabrication of the counter plate. ( b ) Fluttering images of a stand-alone configuration of dimensions 7.5 × 5 cm as captured with a high-speed camera. ( c ) The regime map of the dynamic interaction between a flag and a plate. Full size image Analysis of fluttering behaviour To optimize an electrical output from the contact-separation behaviour of the flag and rigid plate, it is important to understand the detailed dynamic characteristics of flutters. As shown in Fig. 1b , a flexible Au-coated woven flag exhibited oscillations with a node. From the top to the node, where the fluttering amplitude is nearly zero, only a very small-amplitude oscillation arises. Below the node, a travelling wave propagated toward the trailing edge with increasing amplitude. To induce a self-sustained contact-propagation-separation of conductor and dielectric through the high-frequency oscillation of flag flutter, we simply placed the counter plate next to the flag flutter within a critical distance. We then systematically examined the coupled interaction between the flag and the plate by varying the dimensions of the structures (width w and length L ), bending stiffness of the flag B , flag-plate distance d and incoming velocity U . Physical dimensions for the experimental samples are listed in Supplementary Table 1 . The onset velocity for flutter is largely dependent on the bending stiffness, incoming air velocity and the length of the flag. However, the flag-plate distance had a negligible effect on the stability of the flag. Hysteresis was observed for the flutter onset velocity. The fluttering of the flag suddenly arises above a certain critical velocity. However, once fluttering occurs, it continues despite the decrease of air velocity far below the critical value. Bistability was observed between the two critical velocities, where a small external excitation can induce the transition from the stable to fluttering state. The stability boundary can be characterized in a two-dimensional space of dimensionless parameter as shown in Fig. 1c : the nondimensional velocity, , and the dimensionless mass of the flag, m L /( ρwL ), where m L is the mass per unit length of the flag and ρ is the fluid density. The nondimensional velocity is the ratio of the kinetic energy of incoming flow to the elastic energy of the flag. The dimensionless mass is the mass of the flag relative to that of an interacting fluid. Flags with larger dimensionless mass are prone to fluttering at a lower nondimensional velocity due to the destabilizing effects of inertia. In general, by raising the incoming velocity above the stability boundary, the flexible flag begins to flutter in a periodic manner. In the fluttering region in Fig. 1c , we observed two distinct contact-separation modes. The transition from the single-contact mode in region A ( Fig. 1c ) to the double-contact mode in region B ( Fig. 1c ) occurs as the dimensionless mass decreases, which can be tuned by adjusting the length of the flag. This is because of the transition in bending mode of fluttering flag as shown in Supplementary Fig. 1 . As the flag length decreases, the second bending mode is excited, and contact is then likely to occur only at the trailing edge of the flag, resulting in the single-contact mode. As the flag length increases, double-contact behaviour, composed of one contact in the middle of the flag and a second contact at the end of the flag, arises easily because the third bending mode is excited. The transition between the single- and double-contact mode appears when the dimensionless mass ranges from 0.55 to 0.66. This corresponds to the previously reported condition of bending mode transition of single-paper flutter [29] . Furthermore, most flutter experiments have reported that the bending mode transition arises when the dimensionless mass of the flag is in the range of 0.4–0.8 (refs 30 , 31 , 32 ). 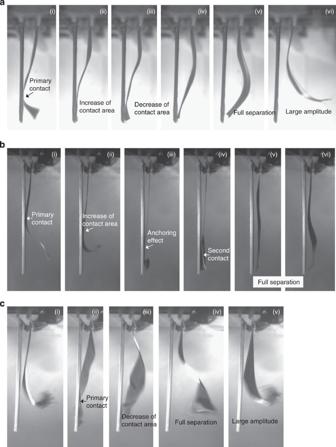Figure 2: Sequential images of contact-separation behaviour. (a) Single-contact mode: fluttering behaviour of a flexible structure with dimensions 7.5 × 5 cm. For (b) double-contact mode and (c) chaotic modes, fluttering behaviour of a flexible structure with dimensions 12 cm (L) × 3 cm (w) was captured by a high-speed camera under a flow velocity of 9.2 ms−1. Figure 2 shows sequential images of the contact-propagation-separation behaviours for the single- and double-contact modes with different flag lengths at a fixed flag-plate separation of 10 mm, captured using a high-speed camera (Photron APX-RS) at the frame rate of 1,500 Hz. The full cycle of contact and separation for each mode is illustrated in Supplementary Fig. 1 for a time interval of 2 ms. In the single-contact mode for the flag of 7.5 × 5 cm in size, the oscillating flag collides with the counter surface with a high kinetic energy due to the large swing amplitude at the edge ( Fig. 2a–i ). The contact surface then increases and decreases again gradually following the travelling wave ( Fig. 2a-ii–iv ). The flag then moves away from the counter plate ( Fig. 2a-v ). The flag finally reaches the maximum amplitude ( Fig. 2a-vi ) and repeats the cycle. In addition, considering the force at the moment of impact between the fluttering flag and the counter surface, the oscillating motion in the single-contact mode is similar to that of a flail with a free-swinging stick or a double pendulum. This motion effectively transforms the angular momentum of the oscillating flag into impact (see details in Supplementary Fig. 2 ). Figure 2: Sequential images of contact-separation behaviour. ( a ) Single-contact mode: fluttering behaviour of a flexible structure with dimensions 7.5 × 5 cm. For ( b ) double-contact mode and ( c ) chaotic modes, fluttering behaviour of a flexible structure with dimensions 12 cm ( L ) × 3 cm ( w ) was captured by a high-speed camera under a flow velocity of 9.2 ms −1 . Full size image On the other hand, in the double-contact mode for flag dimension of 12 × 3 cm, after the first contact occurs ( Fig. 2b-i ), the travelling wave propagates ( Fig. 2b-ii ), which leads to a propagation of the contact area along the wave direction ( Fig. 2b-iii ). A second contact then arises later towards the trailing edge of the flag ( Fig. 2a-iv ), but with a smaller contact strength than the initial contact due to the anchoring effect of the previously contacting surface. The flag then moves away from the counter plate ( Fig. 2a-v,vi ). Another transition can be observed between periodic (regions A and B) and chaotic flutter (region C, Fig. 1c ). The chaotic mode shown in Fig. 2c occurs above a critical nondimensional velocity that is a function of the mass ratio. The chaotic transition boundary can be approximated as . The fluttering motion loses its regularity and becomes random and chaotic. Flutter occurs in a circular or spanwise direction, so that the contact area changes very irregularly. Working principle The electricity generation process in an FTEG is based on the sequence of contact-propagation-separation motion induced by a flutter. It causes gradual increase and decrease of the total contact area via wave propagation, resulting in an electrical signal distinct from what is obtained by a pushing or sliding mode of triboelectric generator. Previous study was shown that the sliding mode is more effective than the pushing mode in terms of the electric signal generation because of the gradual increase in the area at the surface for sliding, which enhances friction [13] , [17] , [33] . From this point of view, electricity generation from an FTEG would be strongly distinguished on the change in effective contact area due to the fluttering behaviour. As shown in Fig. 1a , the configuration of an FTEG is based on the metal-insulator structure and the PTFE, used as an insulator, has a tendency to gain electrons on its surface, and thus will make the surface charged negatively by rubbing the surface (see method). Under no external flow, due to the strong electrostatic attraction, the negatively charged PTFE keeps the good contact with the Au-coated flag. When the flag is blown by the wind, the flag moves backward and forward, following pendulum motion, and there is no electrical charge difference until the moment when contact is made. Right after contact, the propagation process happens and this leads to a gradual increase and decrease in the contact surface, sequentially. That is, a gradual increase in contact surface induces the higher electrical potential on the Au-coated flag and a gradual decrease drops an electrical potential on the Au-coated flag. While the flag periodically approaches the plate, an electrical potential difference between the electrode on the PTFE and the Au-coated flag will occur and a pair of alternating currents is generated. A schematic diagram showing the electrical potential and the working principle of an FTEG is shown in Supplementary Fig. 3 . Electrical characterization of FTEG Voltage and current measurements were carried out under a flow velocity of 7.5 ms −1 for the single- and double-contact modes at a total device size of around 7.5 × 5 cm and 12 × 3 cm, respectively. In the single-contact-separation mode, transferred charges produced an alternating-current output with a short-circuit current ( I sc ) of 25 μA, an open-circuit voltage ( V oc ) of 140 V ( Fig. 3a,b ), and a consecutive contact area of 2 × 5 cm. Scrutinizing the profiles of the electrical signal and the fluttering images, we find that the flag-plate interaction consists of the following steps: a primary contact of the curved area ( Fig. 3c-i, d-i ), an increase in contact area ( Fig. 3c-ii, d-ii ), a decrease in contact area ( Fig. 3c-iii, d-iii ) and eventual separation. These steps are clearly reflected in I sc and V oc . A gradual increase in contact area after primary contact appears to be associated with the distinctive increase in I sc and V oc . A decrease in contact area then appears at separation, which is also evident from the V oc profile. 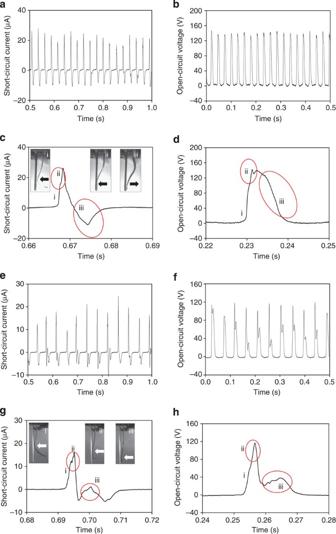Figure 3: Analysis of the electrical signal for each mode. (a–d) Electrical signal of the flutter-driven triboelectric generator under a flow velocity of 7.5 ms−1with dimensions 7.5 × 5 cm. (a) Short-circuit current. (b) Open-circuit voltage. (c) Peak in the profile of short-circuit current. (d) Peak in the open-circuit voltage. (e–h) Electrical signal of the flutter-driven triboelectric generator under a flow velocity of 7.5 ms−1with dimensions 12 × 3 cm. (e) Short-circuit current. (f) Open-circuit voltage. (g) Peak in the short-circuit current. (h) Peak in the open-circuit voltage. Figure 3: Analysis of the electrical signal for each mode. ( a – d ) Electrical signal of the flutter-driven triboelectric generator under a flow velocity of 7.5 ms −1 with dimensions 7.5 × 5 cm. ( a ) Short-circuit current. ( b ) Open-circuit voltage. ( c ) Peak in the profile of short-circuit current. ( d ) Peak in the open-circuit voltage. ( e – h ) Electrical signal of the flutter-driven triboelectric generator under a flow velocity of 7.5 ms −1 with dimensions 12 × 3 cm. ( e ) Short-circuit current. ( f ) Open-circuit voltage. ( g ) Peak in the short-circuit current. ( h ) Peak in the open-circuit voltage. Full size image For the double-contact mode, the two peaks per cycle in I sc and V oc are shown in Fig. 3g,h , which are the results of additional contact at the end of the flexible flag. The fluttering behaviour drives primary contact ( Fig. 3g-i, h-i ), the propagation with an increase in contact area ( Fig. 3g-ii, h-ii ), the second contact at the edge of the flexible structure ( Fig. 3g-iii, h-iii ) and eventual separation. Close investigation of the profile of V oc and I sc finds that the electrical signal of both sequential increase in contact area and the second peak from the edge contact is clearly distinct from that of the single-contact mode. The subsequent change in the contact area due to the travelling wave propagation in fluttering effectively enhances triboelectrification or induces an additional contact mode depending on the flag dimensions. Such propagation is a novel characteristic of an FTEG using a flexible flag. Unlike other types of triboelectric generator, electricity generation in an FTEG is dependent on the polarization magnitude due to the effective contact area and the rate of triboelectric charge separation. In this respect, understanding flutter-induced contact behaviour for different structure dimensions and flow velocities is critical. Performance of an FTEG as a function of flow velocity To investigate the relationship between electric output and fluttering behaviour of a flexible flag as a function of flow velocity, a systematic measurement was performed under flow velocities varying from 7.5 ms −1 to 22 ms −1 . As shown in Fig. 4a , the maximum peak of V oc in the single-contact mode increases with increasing flow velocity and dramatically jumps to the maximum value of 240 V at 22 ms −1 . This result can be explained by an efficient change in surface contact area in the fluttering motion with an increase of flow velocity. At higher wind speeds, a higher fluttering speed results which increases the contact force. Since both the PTFE surface and the woven flexible electrode have a regular micropattern on the surface shown in Fig. 1a , a larger applied force will enhance the microscale contact area between them, resulting in a higher surface charge density [34] , [35] . As the flow velocity increases, the fluttering motion becomes chaotic and an irregular spanwise directional bending of the flutter motion can also be observed, which can increase the effective contact-propagation region unpredictably. This implies that the coupling between flow velocity and fluttering motion may result in an increase of V oc at a higher flow velocity. As shown in Fig. 4b , the peak of I sc increases with increasing wind speed. This occurs because a higher wind speed results in both more transferred charge as discussed before and a higher charge transfer rate with an increase of contact frequency as shown in Fig. 4c . The averaged output current density and power density with variable flow velocities were investigated with a charging rate of a 10-μF capacitor. As shown in Fig. 4d , in the single-contact mode, the charging rate of a 10-μF capacitor increased with flow velocity. 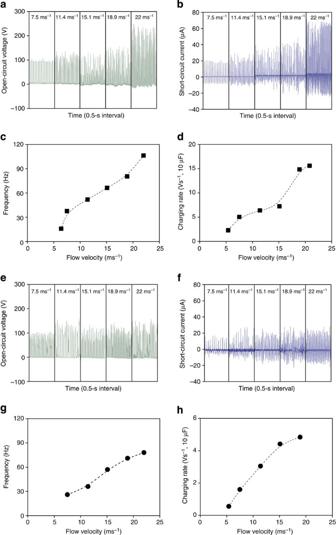Figure 4: Influence of flow velocity on electrical output. (a–d) Electrical output performance of the flutter-driven triboelectric generator with a single-contact configuration. (a) Open-circuit voltage, (b) short-circuit current, (c) frequency of electrical output for single-contact mode and (d) charging rate for a 10-μF capacitor with flow velocities from 7.5 ms−1to 22 ms−1. (e–h) Electrical output performance of the flutter-driven triboelectric generator with a double-contact configuration. (e) Open-circuit voltage, (f) short-circuit current, (g) frequency of electrical output for double-contact mode and (h) charging rate for a 10-μF capacitor with flow velocities from 7.5 ms−1to 22 ms−1. Figure 4: Influence of flow velocity on electrical output. ( a – d ) Electrical output performance of the flutter-driven triboelectric generator with a single-contact configuration. ( a ) Open-circuit voltage, ( b ) short-circuit current, ( c ) frequency of electrical output for single-contact mode and ( d ) charging rate for a 10-μF capacitor with flow velocities from 7.5 ms −1 to 22 ms −1 . ( e – h ) Electrical output performance of the flutter-driven triboelectric generator with a double-contact configuration. ( e ) Open-circuit voltage, ( f ) short-circuit current, ( g ) frequency of electrical output for double-contact mode and ( h ) charging rate for a 10-μF capacitor with flow velocities from 7.5 ms −1 to 22 ms −1 . Full size image In contrast, in the double-contact mode V oc and I sc only slightly increase with flow velocity ( Fig. 4e,f ). Such an effect is because the effective contact area in double-contact mode tends to decrease with increasing flow velocity due to chaotic behaviour, resulting in only a slight increase in electrical output. Although V oc and I sc in double-contact mode are less dependent on flow velocity, the frequency of V oc directly depends on the flow velocity. The charging rate of a 10-μF capacitor increased with increasing flow velocity as shown in Fig. 4g,h . This implies that the frequency of the electrical output plays a dominant role in enhancing the power density of a triboelectric generator system. Durability and efficiency In the FTEG system, the durability of the device will depend on that of the flag material because of the cyclic impact motion. We tested an electrical performance during prolonged fluttering. Prior to the test, the selvage of the flag was sealed with an adhesive to prevent threads from coming loose. The average electrical performance was evaluated by monitoring the time it took to charge a 1,000-μF capacitor to 30 V in every charging cycle. The results indicated that the charging time did not change significantly even after a continuous 12 million flutters while slight damage to the flag around the bottom edge was observed (see Supplementary Fig. 4a ). In addition, a flag contaminated intentionally with dust was employed for the charging test to confirm the reliability in dirty open environments. The charging time with the dust-contaminated flag increased, but after seven charging cycles (about 15min), the charging time recovered significantly to reach ~110% of the charging time of the dust-free flag (see Supplementary Fig. 4b ). We suppose that the high frequency of the oscillating flag would prevent the flag from becoming contaminated by environmental dust as well as acting to remove dust. The electromechanical efficiency of the FTEG can be defined as the ratio of the electric energy generated by a single-plate FTEG to the mechanical energy of the flag. The mechanical energy of the flag can be calculated from the images captured by a high-speed camera at the instant of contact; flag dimensions of 7.5 × 5 cm and a 7.1-ms −1 flow velocity result in a mechanical energy of 0.018 mJ per cycle. The induced electrical energy under the same conditions is 0.0018, mJ at a load of 2 MΩ. The energy conversion efficiency is thus calculated to be 10%. Application of multiple arrays of FTEGs Using a simple dual-plate design with dimensions 7.5 × 5 cm at a 15-ms −1 flow velocity, the electrical signals were obtained as shown in Fig. 5a,b . The frequency of the electrical output reached 158 Hz, and I sc and V oc increased up to 50 μA and 200 V, respectively. The improved frequency and electrical output characteristics imply a larger average system power density, which can be combined with an energy storage system such as capacitors or batteries. For this purpose, the charging time of a 100-μF capacitor to 10 V was compared with different configurations of a single plate (A), a dual plate (B) and a parallel connection of two dual plate with circuit A (C) and circuit B (D) (see Supplementary Fig. 5 ) as shown in Fig. 5c . We see that the charging time decreases from 174 s to 73 s when a dual-plate configuration is used. In the parallel connection, the charging time can be further reduced from 50 s to 37 s by adopting different circuit designs that connect the rectifier to each unit. 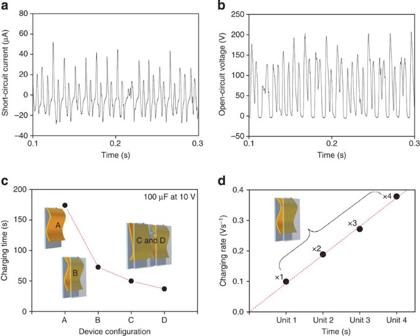Figure 5: Results of electrical measurements for the dual-plate configuration of flutter-driven triboelectric generator. (a) Short-circuit current with dimensions 7.5 × 5 cm at a flow velocity of 15 ms−1. (b) Open-circuit voltage with dimensions 7.5 × 5 cm at a flow velocity of 15 ms−1. (c) Charging time of a 100-μF capacitor to 10 V with a single plate, dual plates and a parallel connection between two dual units at a flow velocity of 15 ms−1. (d) The charging rate increasing with the number of units connected side-by-side and in 2-by-2 arrays at a flow velocity of 15 ms−1. Figure 5d shows that the charging rate increases linearly with the number of units arranged side by side. Figure 5: Results of electrical measurements for the dual-plate configuration of flutter-driven triboelectric generator. ( a ) Short-circuit current with dimensions 7.5 × 5 cm at a flow velocity of 15 ms −1 . ( b ) Open-circuit voltage with dimensions 7.5 × 5 cm at a flow velocity of 15 ms −1 . ( c ) Charging time of a 100-μF capacitor to 10 V with a single plate, dual plates and a parallel connection between two dual units at a flow velocity of 15 ms −1 . ( d ) The charging rate increasing with the number of units connected side-by-side and in 2-by-2 arrays at a flow velocity of 15 ms −1 . Full size image Demonstration in an open environment To demonstrate the performance of an FTEG in an ambient environment, we prepared two types of set-ups, as explained in the following. First, we incorporated an FTEG into a weathercock so that the system can work under the wind of any direction. We observed the fluttering behaviour of the rotatable FTEG (see Supplementary Movie 1 ) and investigated its electrical performance by charging a 10-μF capacitor to 0.5 V with a maximum open-circuit voltage of 100 V and short-circuit current of 12.5 μA ( Fig. 6a ) at an ambient wind velocity of around 3.7–5 ms −1 (3 BF in Beaufort wind force scale). In response to an arbitrary natural wind direction, the rotatable FTEG repositioned itself so that it was parallel to the wind direction. The charging time of the capacitor in an open environment shown in Fig. 6b , and various natural wind speeds result in different charging slopes. Second, a solid, robust of FTEG-packaging module was also designed as shown in Fig. 6c , which enables the FTEG to be securely mounted on the roof of a moving vehicle (see Supplementary Movie 2 ). 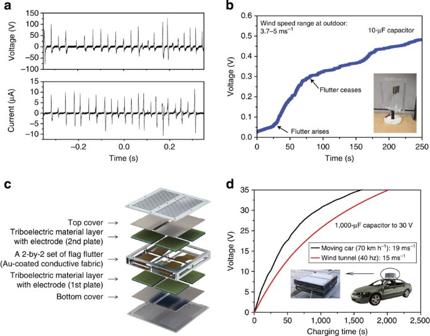Figure 6: Demonstrations of the flutter-driven triboelectric generator (FTEG) in an open environment. Electrical output performance of the rotatable FTEG in an outdoor space: (a) open-circuit voltage (top) and short-circuit current (bottom) at a wind speed of 3.7–5 ms−1. (b) Charging time of a 10-μF capacitor to 0.5 V charged by the rotatable FTEG (inset: image of the rotatable FTEG at a wind speed of 3.7–5 ms−1. SeeSupplementary Fig. 6for a large image). (c) Schematic of the stacked FTEG-packaging module with total eight units. (d) Comparison of the charging times of a 1,000-μF capacitor using a stacked FTEG system when charging on the moving vehicle and when charging in the wind tunnel system. Figure 6d shows the electrical performance of charging a 1,000-μF capacitor to 30 V with the FTEG attached to a car moving at a speed of 70 km h −1 (19 ms −1 ), in comparison with the charging performance within the wind tunnel at 15 ms −1 wind speed. A charging time of 25 min is obtained when the car is travelling at 70 km h −1 . These demonstrations confirmed that the FTEG can operate in an open environment under a variety of wind conditions. Figure 6: Demonstrations of the flutter-driven triboelectric generator (FTEG) in an open environment. Electrical output performance of the rotatable FTEG in an outdoor space: ( a ) open-circuit voltage (top) and short-circuit current (bottom) at a wind speed of 3.7–5 ms −1 . ( b ) Charging time of a 10-μF capacitor to 0.5 V charged by the rotatable FTEG (inset: image of the rotatable FTEG at a wind speed of 3.7–5 ms −1 . See Supplementary Fig. 6 for a large image). ( c ) Schematic of the stacked FTEG-packaging module with total eight units. ( d ) Comparison of the charging times of a 1,000-μF capacitor using a stacked FTEG system when charging on the moving vehicle and when charging in the wind tunnel system. Full size image We have shown that fluttering behaviour can be effectively employed to induce a contact-propagation-separation of a flexible flag and a rigid plate for triboelectrification. The regimes of dynamic interactions including single-contact, double-contact and chaotic modes were identified in a regime map for different flag lengths and flow velocities. Each contact mode resulted in a distinct frequency and amplitude for the electrical output. The single-contact mode exhibited large electrical outputs and high fluttering frequency. With increasing flow velocity, electric performance was enhanced linearly. In the FTEG, the average power density depended on contact force, effective contact area and a type of contact motion including a stable periodic contact and chaotic contact, in addition to the frequency of the electrical output. We demonstrated a self-sustained FTEG with a maximum voltage of 250 V and current of 70 μA at a flow velocity of 22 ms −1 . With a dual-plate FTEG design, the frequency of the electrical performance reached 158 Hz at a flow velocity of 15 ms −1 . This work introduced a new route for triboelectric energy harvesting by utilizing the well-known phenomenon of a fluttering flag, which is a self-sustained motion with extremely high frequency. This FTEG shows excellent electrical performance with a very simple configuration and has the potential for implementation over large areas at low cost. This system can improve electronic performance without size and shape limitations. Fabrication of an FTEG To induce the fluttering behaviour, a conductive, highly flexible, Au-coated woven fabric (80 μm, Solueta SILTEX) was prepared as a flag-type electrode. This was coated with multiple layers of metal electrodes via electroless plating. For the rigid counter plate, the same conductive fabric was placed on the rigid substrate, and a PTFE film (50 μm, 3 M) with adhesive on one side was deposited on top of the electrode as shown in Fig. 1a-iii . The PTFE film acted as a triboelectric active layer with high electron affinity. The conductive woven surface ( Fig. 1a-i ) is composed of tens of microfilaments that are interlaced, and the microtextured surface of the woven fabric can be transferred to the film surface by rubbing ( Fig. 1a-ii ) with high pressure ( Supplementary Fig. 7 ). Experimental set-up for characterization In the typical wind tunnel system, a specific holder was attached to install the FTEG. The prepared flexible electrode and the triboelectric active plate with top and bottom electrodes were placed on the holder with 1-cm separation in accordance with the coupled interaction experiment between the flag and the plate shown in Supplementary Table 1 . Both the top and bottom electrodes were connected to the electrometer (Keithley 6514) to measure the electrical performances including the open-circuit voltage, short-circuit current and capacitor-charging time. The fluttering behaviour of the flag was characterized by capturing the bending motions using a high-speed camera (Photon APX-PS) at a frame rate of 1,500 Hz. How to cite this article: Bae, J. et al. Flutter-driven triboelectrification for harvesting wind energy. Nat. Commun. 5:4929 doi: 10.1038/ncomms5929 (2014).